Identification of a low-spin acylperoxoiron(III) intermediate in bio-inspired non-heme iron-catalysed oxidations Synthetically useful hydrocarbon oxidations are catalysed by bio-inspired non-heme iron complexes using hydrogen peroxide as oxidant, and carboxylic acid addition enhances their selectivity and catalytic efficiency. Talsi has identified a low-intensity g =2.7 electron paramagnetic resonance signal in such catalytic systems and attributed it to an oxoiron(V)-carboxylate oxidant. Herein we report the use of Fe II (TPA*) (TPA*=tris(3,5-dimethyl-4-methoxypyridyl-2-methyl)amine) to generate this intermediate in 50% yield, and have characterized it by ultraviolet–visible, resonance Raman, Mössbauer and electrospray ionization mass spectrometric methods as a low-spin acylperoxoiron(III) species. Kinetic studies show that this intermediate is not itself the oxidant but decays via a unimolecular rate-determining step to unmask a powerful oxidant. The latter is shown by density functional theory calculations to be an oxoiron(V) species that oxidises substrate without a barrier. This study provides a mechanistic scenario for understanding catalyst reactivity and selectivity as well as a basis for improving catalyst design. Non-heme iron complexes have recently emerged as potentially useful oxidation catalysts for the regio- and/or stereoselective functionalization of C–H and C=C bonds with H 2 O 2 as the oxidant [1] , [2] , [3] . These catalysts are inspired by the large family of oxygen activating non-heme iron enzymes that carry out a variety of oxidative transformations in metabolically important molecules [4] , [5] , [6] . The bio-inspired complexes belonging to this class are typically supported by tetradentate N4 ligands ( Fig. 1a ) and have an iron center with two cis -labile coordination sites at which to activate the H 2 O 2 for reactions that exhibit high retention of configuration [1] , [2] , [3] . Their catalytic activity and selectivity are further enhanced by the addition of acetic acid to the reaction mixture, leading to predictable regio- and stereoselectivity in the oxidation of particular aliphatic C–H bonds in complex organic molecules, as demonstrated by White for (+)-artemisinin and (−)-dihydropleuromutilone [7] , [8] . Highly enantioselective olefin epoxidation reactions can also be achieved [9] , [10] , [11] , [12] . 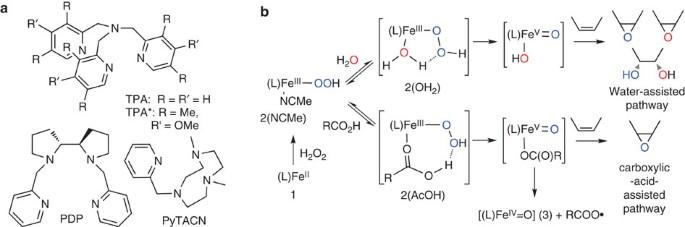Figure 1: Proposed mechanisms for bio-inspired non-heme iron catalysts in olefin oxidations. (a) Tetradentate ligands used in non-heme iron catalysts. (b) Proposed mechanisms for the activation of hydrogen peroxide by non-heme iron oxidation catalysts with the assistance of water or carboxylic acids. Complexes1–3designate species with L=TPA, while1*–3*correspond to species with L=TPA*. Figure 1: Proposed mechanisms for bio-inspired non-heme iron catalysts in olefin oxidations. ( a ) Tetradentate ligands used in non-heme iron catalysts. ( b ) Proposed mechanisms for the activation of hydrogen peroxide by non-heme iron oxidation catalysts with the assistance of water or carboxylic acids. Complexes 1 – 3 designate species with L=TPA, while 1* – 3* correspond to species with L=TPA*. Full size image The selectivity exhibited by these reactions strongly implicates a metal-based species, rather than HO·, as the oxidant generated by the reaction of the iron complex with H 2 O 2 (ref. 13 ) In early studies, Que and co-workers observed the generation of a (TPA)Fe III –OOH intermediate upon reaction of the [(TPA)Fe II ] catalyst ( 1 ) with excess H 2 O 2 at −40 °C in CH 3 CN solvent, as well as label incorporation from H 2 18 O into the oxidation products [14] , [15] . These results led to postulation of a mechanism that involves heterolytic cleavage of the O–O bond in the Fe III –OOH intermediate that was promoted by bound water to form a Fe V (O)(OH) oxidant ( Fig. 1b ). This hypothesis has received recent support from kinetic studies demonstrating both an accelerative effect of added water and a significant H 2 O/D 2 O kinetic isotope effect (KIE) on both the decay rate of the Fe III –OOH intermediate and the rate of product formation [16] . Direct spectroscopic evidence for the putative Fe V (O)(OH) oxidant was obtained by Costas and Cronin from variable temperature electrospray mass spectrometric experiments in studies of their [(PyTACN)Fe II (OTf) 2 ] catalyst [17] . To account for the effect of the acetic acid additive first observed by White [18] , Mas-Balleste and Que modified the proposed water-assisted mechanism into a carboxylic-acid-assisted version that generates an Fe V (O)(OAc) oxidant ( Fig. 1b ) [19] . Such an oxidant would be consistent with the observed increase in epoxide selectivity at the expense of cis -diol formation in the oxidation of olefins. The involvement of the Fe V (O)(OAc) oxidant was also supported by the formation of a minor cis- hydroxyacetoxylated product in olefin oxidation by Fe(TPA) in the presence of acetic acid [20] as well as the observed decay of the Fe III –OOH intermediate in the presence of a carboxylic acid to the corresponding Fe IV (O) species 3 and a carboxyl radical, which was found to occur in competition with the formation of olefin oxidation products when olefin substrate was present [19] . Talsi and co-workers claimed to have observed the putative Fe V (O)(O 2 CR) oxidant, as evidenced by a novel S =½ electron paramagnetic resonance (EPR) signal at g =2.71, 2.42 and 1.53, in the reaction of 40-mM 1 in 1:1.7 CH 3 CN/CH 2 Cl 2 with either 30% H 2 O 2 /AcOH, peracetic acid or m -chloroperbenzoic acid ( m CPBA) at −60 °C (ref. 21 ). The EPR signal exhibited a self-decay rate of 1.6(2) × 10 −3 s −1 at −70 °C, which increased fivefold upon addition of 12 equiv. cyclohexene with concomitant formation of cyclohexene oxide. However, EPR quantification showed that the g =2.7 species was formed in only 7% yield, and no additional spectroscopic characterization to support the claimed Fe V oxidation state assignment was reported. Subsequently, similar EPR features were found for related non-heme iron catalysts [9] , [12] , [22] , [23] , [24] . Here we report reaction conditions that increase the yield of the g =2.7 intermediate to 50%, paving the way for its characterization by ultraviolet–visible, Mössbauer, resonance Raman and electrospray mass spectrometric methods. Taken together, our data show that the intermediate is in fact a low-spin acylperoxoiron(III) complex that undergoes rate determining O–O bond cleavage to unmask the oxidant that carries out substrate oxidation. Generation of intermediates 4 and 4* Our attempts to characterize the g =2.7 species started with the introduction of excess H 2 O 2 (70%) to a CH 3 CN solution of 1 ( Fig. 1a , L=TPA) in the presence of excess AcOH at −40 °C. This reaction afforded a species that exhibits an absorbance maximum at 460 nm ( Supplementary Fig. 1 ), a brown chromophore that is distinct from the purple chromophore obtained in the absence of AcOH and associated with the Fe III –OOH intermediate 2 ( λ max 540 nm) [25] . The brown intermediate, designated as 4 , has a lifetime of only 5 min at −40 °C and decays to the corresponding (TPA)Fe IV (O) species 3 ( λ max =720 nm) in about 70% yield, while 2 persists for up to 3 h under similar conditions [15] , [16] , indicating that 4 is significantly more reactive than the Fe III –OOH complex 2 . Even more importantly, the EPR features obtained for a frozen CH 3 CN solution of 4 are identical to those reported by Talsi and assigned to an Fe V (O) species ( Supplementary Fig. 2 ) [21] , [22] . Simulation of the EPR signals of 4 using the SpinCount software [26] shows that this species is formed in ~20% yield, an amount that is higher than that reported by Talsi, but still not high enough to determine its oxidation state reliably via Mössbauer spectroscopy. To increase the fraction of the g =2.7 intermediate in our samples required extending the lifetime of the intermediate. This goal was achieved by replacing TPA with its more electron donating variant TPA* ( Fig. 1a ), an approach that previously enabled us to generate highly reactive (μ-oxo)diiron complexes [27] , [28] . First, we found 1 and 1* (Fe II (TPA*)) to have comparable catalytic alkane and olefin oxidation reactivity ( Supplementary Table 1 ). Next we demonstrated that addition of 10 equiv. 70% H 2 O 2 to a 0.5-mM 1* in CH 3 CN in the presence of 200 equiv. AcOH at −40 °C also produced a 460-nm chromophore ( Fig. 2 ), designated 4* . This species had at least twice the intensity of that produced from 1 and was distinct from the purple Fe III –OOH chromophore 2*(OH 2 ) ( λ max 510 nm) generated in the absence of AcOH ( Supplementary Fig. 3 ). In this case, the 460-nm intermediate persisted in a steady state phase before undergoing rapid exponential decay ( k decay =0.019 s −1 ) to give rise to the Fe IV =O complex 3* ( λ max 720 nm) in ~70 % yield. Intermediate 4* also formed in comparable yields in the reactions of 1* with peracetic acid or m CPBA at −40 °C ( Supplementary Fig. 4 ). In the case of peracetic acid, 4* decayed to 3* as observed for the H 2 O 2 /AcOH combination. However, for m CPBA, the intermediate analogous to 4* evolved into a different chromophore with a λ max at 560 nm that was associated with an iron(III)-salicylate complex derived from self-hydroxylation [29] . 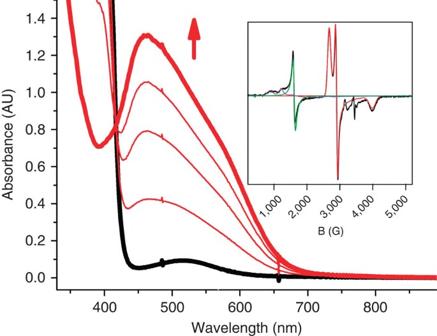Figure 2: Characterization of 4* by UV-vis and electron paramagnetic resonance spectroscopy. Ultraviolet visible spectral evolution of intermediate4*(red trace) upon addition of 10 equiv. 70% H2O2at −40 °C to 0.5-mM1*(L=TPA*, Figure 1a) (black trace) in CH3CN in the presence of 200 equivalents of acetic acid. Inset: X-band electron paramagnetic resonance spectrum (black line) of intermediate4*in CH3CN. The red line shows anS=1/2 spectral simulation for4*usinggx=1.72,gy=2.38 andgz=2.58 with a line width assuming a Gaussian distribution ofg-values withσ(gx,y,z)=(0.04; 0.02; 0.045). The simulation represents 47% of the Fe in the sample. The remaining signals derive from two high-spin (S=5/2) ferric species, which together represent ca. 35% of total Fe; details can be found in the Supporting Information. Conditions: 9.64 GHz frequency, 20 μW microwave power, 1 mT modulation, Temperature=10 K. Figure 2: Characterization of 4* by UV-vis and electron paramagnetic resonance spectroscopy. Ultraviolet visible spectral evolution of intermediate 4* (red trace) upon addition of 10 equiv. 70% H 2 O 2 at −40 °C to 0.5-mM 1* (L=TPA*, Figure 1a) (black trace) in CH 3 CN in the presence of 200 equivalents of acetic acid. Inset: X-band electron paramagnetic resonance spectrum (black line) of intermediate 4* in CH 3 CN. The red line shows an S =1/2 spectral simulation for 4* using g x =1.72, g y =2.38 and g z =2.58 with a line width assuming a Gaussian distribution of g -values with σ ( g x , y , z )=(0.04; 0.02; 0.045). The simulation represents 47% of the Fe in the sample. The remaining signals derive from two high-spin (S=5/2) ferric species, which together represent ca. 35% of total Fe; details can be found in the Supporting Information. Conditions: 9.64 GHz frequency, 20 μW microwave power, 1 mT modulation, Temperature=10 K. Full size image Kinetics studies Intermediate 4* can also be generated at −40 °C in the presence of olefins ( Fig. 3 ). When 1* was reacted with H 2 O 2 /AcOH in the presence of 250 equiv. 1-octene, the characteristic band of 4* at 460 nm formed rapidly, persisted in a steady state phase, and underwent exponential decay upon depletion of H 2 O 2 with a first order rate constant of 0.018(3) s −1 . In a parallel experiment, GC product analysis was carried out on aliquots of the reaction mixture quenched at −40 °C, and the formation of 1,2-epoxyoctane was monitored as a function of time. Notably, formation of epoxide occurred only after the 460-nm species was generated and ceased upon complete decay of 4* . The product was formed linearly versus time at a rate of 0.017(3) mM s −1 , which upon division by the catalyst concentration gives a rate constant of 0.017(3) s −1 for product formation, in excellent agreement with the rate constant for 4* decay. Furthermore, the rate of 4* decay was found to be independent of the amount of substrate present (0–250 equiv.) as well as the nature of the substrate (1-octene, cyclooctene or 2-heptene) ( Supplementary Table 2 ). This kinetic behaviour is similar to that of the closely related (TPA)Fe III –OOH species 2 in olefin oxidation reactions, where 2 was shown to undergo water-assisted rate-determining O–O bond heterolysis to afford an Fe V (O)(OH) oxidant [16] . 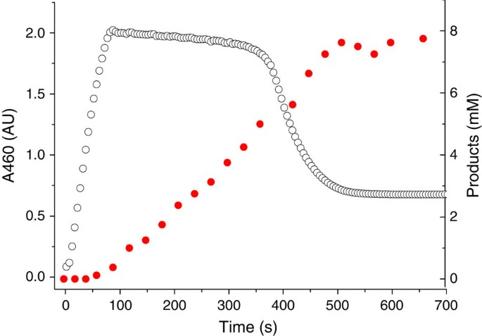Figure 3: Time course for the evolution of4*in the catalytic oxidation of 1-octene. Monitoring the A460 value corresponding to intermediate4*(black open circles) as a function of time in the oxidation of 1-octene (250 eq) with1*(1.0 mM) and 20 eq. 70% H2O2at −40 °C. Parallel monitoring of the epoxide product (red-filled circles) by gas chromatographic analysis of the reaction aliquots quenched at −40 °C. Figure 3: Time course for the evolution of 4* in the catalytic oxidation of 1-octene. Monitoring the A460 value corresponding to intermediate 4* (black open circles) as a function of time in the oxidation of 1-octene (250 eq) with 1* (1.0 mM) and 20 eq. 70% H 2 O 2 at −40 °C. Parallel monitoring of the epoxide product (red-filled circles) by gas chromatographic analysis of the reaction aliquots quenched at −40 °C. Full size image Additional kinetic data were obtained to gain insight into how the decay of 4* differs from the decay of 2 . The decay of intermediate 2 ( OH 2 ) in the corresponding 1 -catalysed oxidation of olefins in the absence of acetic acid was found to be accelerated with increasing water concentration and to exhibit a KIE value of 2.5 when H 2 O was substituted with D 2 O (ref. 16 ). These observations support the proposed water-assisted mechanism where rate determining heterolytic O–O bond cleavage is facilitated by the adjacent water ligand ( Fig. 1b ). In contrast, for the catalytic oxidation in the presence of acetic acid, the decay rate of the 460-nm intermediate 4* was not affected by AcOH concentration, nor was a KIE observed when AcOH was replaced by AcOD ( Supplementary Table 2 ). Analysis of the temperature dependence of 4* decay ( Supplementary Fig. 5 ) gave Eyring activation parameters of ΔH ‡ =16(1) kcal mol −1 and ΔS ‡ =3(5) cal K −1 mol −1 , which were quite distinct from those for the decay of 2 ( OH 2 ). While 4* decay has an activation enthalpy 5 kcal/mol higher than that for 2 ( OH 2 ) decay, its activation entropy is essentially zero compared to a value of −23(5) cal K −1 -mol −1 for 2 ( OH 2 ) decay. These values correspond to a free energy of activation of 15.5 kcal mol −1 at 233 K for 4* decay, which is 0.7 kcal mol −1 smaller than that for 2 ( OH 2 ) decay, accounting for the 10-fold faster decay rate of 4* . The rate of 4* decay extrapolated from the Eyring plot to −70 °C of 0.00067, s −1 is in reasonable agreement with the rate of 0.0017, s −1 obtained by Talsi for the decay of the EPR signal of 4 (ref. 21 ); the latter would be expected to be somewhat faster due to the lower basicity of TPA. However, contrary to Talsi’s observations, we did not observe an accelerative effect of the addition of substrate on the decay of 4* , consistent with our hypothesis that 4* is not the actual oxidant in these reactions but its precursor ( Supplementary Table 2 ). Taken together, these observations demonstrate that 4* is a kinetically competent intermediate for mediating olefin oxidation, and thus the two oxidising equivalents required for this conversion must be stored in 4* . Spectroscopic characterization of 4* Various spectroscopic techniques were thus applied to gain insight into the composition and electronic structure of 4* . To establish its elemental composition, electrospray ionization mass spectrometry (ESI-MS) experiments were carried out at −40 °C on 4* . Although our attempts on 4* generated from the reaction of 1* with H 2 O 2 /AcOH or peracetic acid at −40 °C were unsuccessful, the experiment with m CPBA revealed two predominant mass envelopes at m / z =345.6167 and 690.1944 ( Fig. 4 ). The m / z =690.1944 peak arises from [(TPA*)Fe III (5-Cl-salicylate)] + (calcd for C 34 H 39 ClFeN 4 O 6 =690.1908), which is a byproduct that results from self-hydroxylation of the m CPBA ligand, as previously observed in the reaction of 1 with m CPBA [29] . On the other hand, the m / z =345.6167 peak has a value and isotope distribution pattern corresponding to an elemental composition of [C 34 H 40 ClFeN 4 O 6 ] 2+ (calcd 345.5988). This peak can be associated with the transient 460-nm chromophore, as it was not present in ESI-MS spectra obtained after the 460-nm chromophore had decayed. Its elemental composition and transient nature suggest a formulation as either the acylperoxoiron(III) species [(TPA*)Fe III (O 3 CC 6 H 4 Cl)] 2+ or the subsequent O–O cleaved species [(TPA*)Fe V (O)(O 2 CC 6 H 4 Cl)] 2+ proposed by Talsi [21] . To clarify this ambiguity, additional experiments were performed to assign the iron oxidation state and determine whether an O–O bond was present. 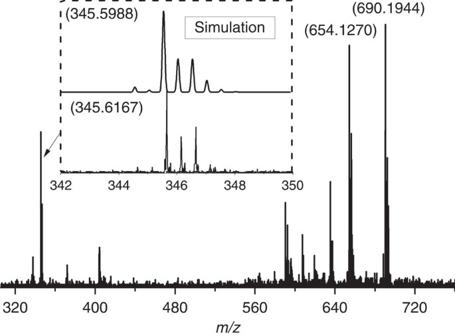Figure 4: Characterization of4*by high-resolution mass spectrometry. Electrospray ionization mass spectrometric characterization of the reaction mixture of1*and excess meta-chloroperoxybenzoic acid in CH3CN at −40 °C revealing a peak atm/z=345.6167 that has a mass and isotope distribution pattern consistent with4*(calcd for [C34H40ClFeN4O6]2+=345.5988). Peaks atm/z654.1270 and 690.1944 can, respectively, be assigned to [(TPA*)FeIII(Cl)ClO4]+(calcd for C27H36Cl2FeN4O7=654.1311) and [(TPA*)FeIII(5-Cl-salicylate)]+(calcd for C34H39ClFeN4O6=690.1908). Figure 4: Characterization of 4* by high-resolution mass spectrometry. Electrospray ionization mass spectrometric characterization of the reaction mixture of 1* and excess meta-chloroperoxybenzoic acid in CH 3 CN at −40 °C revealing a peak at m / z =345.6167 that has a mass and isotope distribution pattern consistent with 4* (calcd for [C 34 H 40 ClFeN 4 O 6 ] 2+ =345.5988). Peaks at m / z 654.1270 and 690.1944 can, respectively, be assigned to [(TPA*)Fe III (Cl)ClO 4 ] + (calcd for C 27 H 36 Cl 2 FeN 4 O 7 =654.1311) and [(TPA*)Fe III (5-Cl-salicylate)] + (calcd for C 34 H 39 ClFeN 4 O 6 =690.1908). Full size image The 460-nm intermediate, 4* , exhibits an EPR spectrum with g -values at g =2.58, 2.38 and 1.72 ( Fig. 2 , inset) that represents 47% of the Fe in the sample based on a SpinCount simulation [26] , as indicated by the red line. The fraction of Fe represented by this species is 3–7 times higher than that reported for the g =2.7 species by Lyakin et al . [21] , [22] There are also two additional S =5/2 signals that arise from high-spin ( S =5/2) iron(III): a major component (purple curve, ≈30% of Fe) that originates from the upper Kramers doublet of a species with D ≈−0.8 cm −1 and E / D ≈0.10 and a minor fraction (green curve, ~5 % of Fe) with E / D ≈1/3 that gives rise to the resonance at g =4.3. The S =1/2 EPR signals of the 460-nm intermediates generated from the reaction of 1* with peracids have g -values and intensities comparable with those shown in the inset of Fig. 2 ( Supplementary Fig. 4 ) [24] . 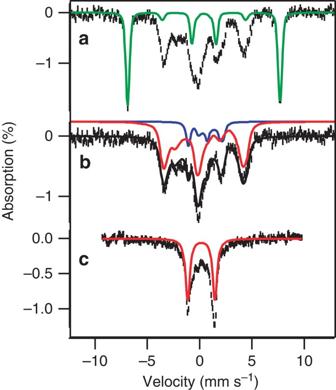Figure 5: Mossbauer spectroscopic characterization of 4* in acetonitrile. (a) Spectrum recorded at 4.2 K in a parallel applied field of 8.0 T. The green line is a theoretical curve representing 35% of the iron belonging to a high-spin FeIIIspecies withD=−0.8 cm−1andE/D=0.10 (see Supplementary Information). (b) 8.0 T spectrum of intermediate4*obtained from (a) by subtracting the contribution of the high-spin FeIIIspecies. The red curve, representing 50% of iron, is a simulation for4*using equation (1) and the parameters:gx,y,z=(1.72, 2.38, 2.58),Ax,y,z/gnβn=(−45, +19, +31) T, ΔEQ=+2.6 mm s−1,η=−6, δ=0.23 mm s−1. The blue curve is attributed to a diiron(III) contaminant (≈12% of iron, see SI). The black line is the sum of the red and blue curves. Additional 4.2 K spectra recorded at 0.1, 2.0 and 5.0 T are shown in Supplementary Information. (c) Zero field spectrum recorded at 160 K. The doublet outlined in red is attributed to4*. The absorption in the center belongs to the diferric species (blue line inb) and in part to mononuclear high-spin FeIIIundergoing intermediate relaxation. Spectra were simulated using the software WMOSS. Figure 5 shows Mössbauer spectra of the same sample as used for the EPR spectrum of Fig. 2 , inset. Additional spectra recorded in variable applied magnetic fields, B, are shown and discussed in Supplementary Fig. 6 . The green line in the 8.0 T spectrum of Fig. 5a , is a spectral simulation (normalized to represent 35% of Fe) for the two high-spin Fe III species; we comment in Supplementary Note 1 why these species are indistinguishable at 8.0 T. Subtracting the simulated spectrum from the raw data yields the spectrum in Fig. 5b that, except for a small diamagnetic contaminant (12% of Fe, blue line, see Supplementary Fig. 6 and note 1 ), represents the S =1/2 species 4* observed in a parallel applied field of 8.0 T. At 4.2 K the spin system of the S =1/2 species is in the slow relaxation regime and its spectra exhibit paramagnetic hyperfine structure. At T =160 K, however, the electronic spin relaxes fast so that the magnetic hyperfine interactions are averaged out, yielding a quadrupole doublet for the S =1/2 species ( Fig. 5c , red line) with splitting Δ E Q =2.60±0.05 mm s −1 and isomer shift δ=+0.17±0.03 mm s −1 . (After a correction for the second-order Doppler shift, the latter value translates to δ≈+0.23 mm s −1 at 4.2 K.) The value of δ falls squarely into the range reported for related non-heme low-spin Fe III -peroxo complexes [30] ( Table 1 ) and is about 0.2 mm s −1 higher than that found for the ferryl complex [Fe IV (O)(TPA)(NCCH 3 )] 2+ (ref. 31 ). For comparison, the δ value for [Fe V (O)(TAML)] − , the bona fide S=½ Fe V =O complex reported by Tiago de Oliveira et al. has δ=−0.42±0.03 mm s −1 (ref. 32 ) (the δ value of the other established Fe V =O complex, [(TMC)Fe V (O)(NR)] + , has a more positive δ value, due to the presence of a trans O=Fe=NR unit) [33] . Figure 5: Mossbauer spectroscopic characterization of 4* in acetonitrile. ( a ) Spectrum recorded at 4.2 K in a parallel applied field of 8.0 T. The green line is a theoretical curve representing 35% of the iron belonging to a high-spin Fe III species with D =−0.8 cm −1 and E / D =0.10 (see Supplementary Information). ( b ) 8.0 T spectrum of intermediate 4* obtained from ( a ) by subtracting the contribution of the high-spin Fe III species. The red curve, representing 50% of iron, is a simulation for 4* using equation (1) and the parameters: g x , y , z =(1.72, 2.38, 2.58), A x , y , z / g n β n =(−45, +19, +31) T, Δ E Q =+2.6 mm s −1 , η =−6, δ=0.23 mm s −1 . The blue curve is attributed to a diiron(III) contaminant (≈12% of iron, see SI). The black line is the sum of the red and blue curves. Additional 4.2 K spectra recorded at 0.1, 2.0 and 5.0 T are shown in Supplementary Information. ( c ) Zero field spectrum recorded at 160 K. The doublet outlined in red is attributed to 4* . The absorption in the center belongs to the diferric species (blue line in b ) and in part to mononuclear high-spin Fe III undergoing intermediate relaxation. Spectra were simulated using the software WMOSS. Full size image Table 1 Vibrational and Mössbauer parameters for various non-heme peroxoiron(III) complexes. Full size table We have analysed the 4.2 K spectra of 4* using the S =1/2 spin Hamiltonian where and g is the electronic g-tensor and A the magnetic hyperfine tensor. H Q describes the interaction of the nuclear quadrupole moment Q with the electric field gradient (EFG) tensor (principal components V ii ); is the asymmetry parameter. For the analysis, we have assumed that all tensors share a common principal axis system, defined by the principal g -values of the S =1/2 species, g x , y , z =1.72, 2.38 and 2.58. The best match to the intensities is obtained by assuming that 4* represents 50% of the total Fe, a value in excellent agreement with the EPR quantification (47%). The solid red lines in Fig. 5 and Supplementary Fig. 6 are theoretical curves generated from equation (1) for the parameters listed in the caption of Fig. 5 . We wish to comment on a few points. The magnetic splittings of the S =1/2 species are controlled by the internal magnetic field , where ‹ S › is the expectation value of the electronic spin. The anisotropy of g imposes a directional preference (the z direction) on ‹ S ›, a fact which allowed us to establish a spatial correlation between the g , A and EFG tensors. The analysis establishes clearly the signs of the three A-tensor components, and these signs are readily rationalized by analysing the data in the framework of the ( t 2 g ) [5] hole model for low-spin Fe III introduced by Griffith [34] and amended for Mössbauer analysis by Oosterhuis and Lang [35] . Analysis of the g -values in this model reveals that the ground state of the S =1/2 species is predominantly a d yz hole (orbital displayed in Fig. 7). For this state the largest EFG component would be negative and along x , just as observed. (Note: the quoted experimental Δ E Q =+ 2.6 mm s −1 , η =−6 corresponds to Δ E Q =−2.6 mm s −1 , η =0.43 when the EFG is quoted in the conventional frame of the Mössbauer literature, x ′, y ′, z ′, for which | V z ′ z ′ |≥| V y ′ y ′ |≥ | V x ′ x ′ |). The Fermi contact term (scaling factor κ ), the spin dipolar term and the orbital term (which is roughly proportional to g x –2) all have a negative contribution to A x , rationalizing why A x is negative and large. In contrast, the spin-dipolar and (large) orbital contributions along z are positive, yielding a positive A z . Using the model of Oosterhuis and Lang [35] implemented in SpinCount [26] , we obtained Δ=1,015 cm −1 and V =1,157 for the tetragonal and rhombic crystal field splittings, respectively (using λ ≈380 cm −1 for the spin-orbit coupling constant). Using the scaling factors P =2 g n β n ‹ r −3 ›=85 MHz and κ =0.35 (see equation (10) in ref. 35 ), we obtained for the A-tensor components A x , y , z / g n β n =(−44, +20, +31) T, which in sign and magnitude are in excellent agreement with the experimental data ( A x , y , z / g n β n =(−45, +19, +31) T). Thus 4* is definitively a low-spin iron(III) complex. The Mossbauer assignment of 4* as a low-spin iron(III) species and the requirement that 4* must have the two oxidising equivalents to carry out olefin epoxidation lead us to propose 4* as a low-spin acylperoxoiron(III) complex. This assignment is supported by resonance Raman experiments. With 457.9-nm excitation, resonance-enhanced features at ca. 490, 600, 800, 1,300 and 1,700 cm −1 were observed for 4* samples generated with H 2 O 2 /AcOH or m CPBA ( Fig. 6 ). The peaks observed at 600 and 800 cm −1 match well with the two features observed for S =½ [Fe III (L)(OOH)] 2+ complexes, which have been assigned to v (Fe–O) and v (O–O) modes, respectively, by 18 O labelling ( Table 1 ) [4] . Corresponding modes were found at 547 and 884 cm −1 for S =5/2 [Fe III (qn) 2 (OOCO 2 )] − (qn=quinaldate), the only non-heme iron(III) species with an acylperoxo-like ligand to have been characterized by resonance Raman spectroscopy [36] . The lower v (O–O) frequency for 4* compared with that of [Fe III (qn) 2 (OOCO 2 )] − results from the difference in spin states, as previously shown for other non-heme iron-peroxo complexes ( Table 1 ) [4] , [37] . Notably, 4* also exhibits resonance enhanced features at ca. 1,300 and 1,700 cm −1 , which have not been reported thus far for other non-heme iron(III)-peroxo complexes ( Table 1 ). However, similar high frequency modes were observed at 1,298 and 1,744 cm −1 in the Fourier transform infrared spectrum of [Fe III (TPPP)(O 2 C(O)C 6 H 4 -3-Cl)] (TPPP=5,10,15,20-tetrakis(2,4,6-triphenylphenyl)porphyrinato) [38] and can be associated with deformations of the acylperoxo group. Thus the 460-nm chromophore of 4* arises from an acylperoxo-to-iron(III) charge transfer transition. 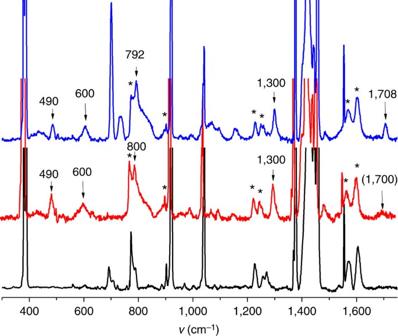Figure 6: Resonance Raman spectroscopic characterization of4*. Spectra (λex=457.9 nm, 40 μW) of frozen samples of1*in CH3CN (black, bottom) and4*prepared from1*and H2O2/AcOH (red, middle) ormCPBA (blue, top). Peaks present in the starting complex1*are marked with an asterisk, while major signals associated with4*are labelled with their frequencies. Figure 6: Resonance Raman spectroscopic characterization of 4* . Spectra ( λ ex =457.9 nm, 40 μW) of frozen samples of 1* in CH 3 CN (black, bottom) and 4* prepared from 1* and H 2 O 2 /AcOH (red, middle) or m CPBA (blue, top). Peaks present in the starting complex 1* are marked with an asterisk, while major signals associated with 4* are labelled with their frequencies. Full size image DFT calculations The assignment of 4* as a low-spin acylperoxoiron(III) species is supported by density functional theory (DFT) calculations. Its geometry optimized structure shown in Fig. 7 (Cartesian coordinates listed in Supplementary Table 3 ) shows a bidentate acylperoxo ligand with the peroxo group bound trans to the tertiary amine and gives calculated Mössbauer parameters (Δ E Q =−2.48 mm s −1 , η =0.20 and δ=0.20 mm s −1 ) that are in excellent agreement with the experimental results (Δ E Q =−2.6 mm s −1 , η =0.43 (quoted in the conventional frame of the EFG tensor) and δ=0.23 mm s −1 ). The calculated EFG tensor also allows us to correlate the axes of the spin Hamiltonian of equations 1 and 2 to the calculated structure. Experimentally, the largest (and negative) component of the EFG tensor is V xx , so V xx , and consequently g x =1.72, are along the acyl oxygen-Fe-N pyr axis. 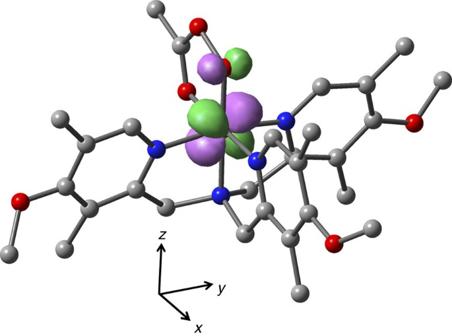Figure 7: DFT geometry optimization of the low-spin acylperoxoiron(III) intermediate4*. The geometry optimization was performed using the Gaussian 09 software and B3LYP/ 6-311G. Hydrogen atoms have been omitted for clarity. Element colours are: red, oxygen; blue, nitrogen; gray, carbon; pink, iron. Shown in magenta/green is the LUMOdyz(β) molecular orbital (representing the hole in the Griffith model). The indicated coordinate axes are the same as those ofSupplementary Table 4; however,xandywere interchanged so thatVxxof equations 1 and 2 correspond toVxxof the calculated EFG, correlating the DFT structure with the spin Hamiltonian. Figure 7: DFT geometry optimization of the low-spin acylperoxoiron(III) intermediate 4* . The geometry optimization was performed using the Gaussian 09 software and B3LYP/ 6-311G. Hydrogen atoms have been omitted for clarity. Element colours are: red, oxygen; blue, nitrogen; gray, carbon; pink, iron. Shown in magenta/green is the LUMO d yz ( β ) molecular orbital (representing the hole in the Griffith model). The indicated coordinate axes are the same as those of Supplementary Table 4 ; however, x and y were interchanged so that V xx of equations 1 and 2 correspond to V xx of the calculated EFG, correlating the DFT structure with the spin Hamiltonian. Full size image Additional DFT calculations have been carried out to gain insight into the mechanism of the Fe II (TPA)/H 2 O 2 /AcOH catalytic reaction. These calculations find acylperoxoiron(III) species 4 to be a relatively stable intermediate, in general agreement with results previously reported in DFT calculations for the Fe II (PDP)/H 2 O 2 /AcOH system [39] , but there are some differences ( Fig. 8a and Supplementary Fig. 7 ). 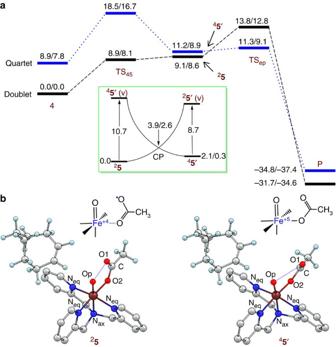Figure 8: DFT energy profiles for cyclooctene epoxidation by4with H2O2and acetic acid. (a) Energy profiles (in kcal mol−1) for cyclooctene epoxidation with energies calculated at the B3LYP/def2-TZVPP//TZVP(Fe,N,O)-6-31G**(H,C) level. The relative energies are reported as zero-point energy (ZPE) corrected energy/free energy values, respectively. Box: schematic plot of the crossing point (CP) between25and45′as well as their vertical transition species25(v) and45′(v). (b) Calculated structures for25and45′prior to attack of cyclooctene substrate with H-atoms on the TPA ligand omitted for clarity. Figure 8a shows the free energy profile for the conversion of 4 to a higher valent species. Intermediate 4 is found to have a doublet ground state and is hereafter designated as 2 4 . Our calculations show that direct reaction of 2 4 with cyclooctene has a barrier of roughly 28 kcal mol −1 ( Supplementary Figs 8–11 and Supplementary Tables 4–6 ), making it unlikely that it is the actual oxidant. Instead, 2 4 undergoes O–O bond cleavage to afford either [(TPA)Fe IV (O)(·OC(O)CH 3 )] ( 5 ) or [(TPA)Fe V (O)(OC(O)CH 3 )] ( 5′ ), which lie at higher energy by 9.1 and 11.5 kcal mol −1 (or 8.6 and 8.9 kcal mol −1 , after considering the entropy contribution) and, respectively, have doublet and quartet spin states; hence they are designated as 2 5 and 4 5′ , respectively ( Table 2 ). Although 2 5 is slightly more stable than 4 5′ , the former can also be excluded as the oxidant because it encounters a substantial barrier for cyclooctene epoxidation and readily reverts to 2 4 without a barrier. In contrast, the perferryl species 4 5′ epoxidises cyclooctene without any barrier, making it a very powerful oxidant. The free energy barrier for the formation of 4 5′ from 2 4 should consist of the barrier (~9 kcal mol −1 ) for O–O bond cleavage from 2 4 to 2 5 and the energy associated with the spin crossover from 2 5 to 4 5′ , which can be estimated from the spin crossover energy diagram shown in Fig. 8 (box), along with the vertical energy gaps between the species. Assuming that the spin crossover probability is unity, then the incremental barrier for this step would simply be the height of the crossing point for the 2 5 to 4 5′ crossover, which depends on the nature of the two curves [40] . If we assume the two curves behave like parabolas, as in Marcus electron transfer theory, then the height of the crossing point will be about 2.6/3.9 kcal mol −1 (using zero-point energy corrected values/free energy values) relative to 2 5 , thus making 13.8/12.9 kcal mol −1 the total zero-point energy-corrected/free energy barriers for epoxidation. This calculated value is in reasonable agreement with the value of 16 kcal mol −1 we have determined experimentally for the decay of 2 4 . Figure 8: DFT energy profiles for cyclooctene epoxidation by 4 with H 2 O 2 and acetic acid. ( a ) Energy profiles (in kcal mol −1 ) for cyclooctene epoxidation with energies calculated at the B3LYP/def2-TZVPP//TZVP(Fe,N,O)-6-31G**(H,C) level. The relative energies are reported as zero-point energy (ZPE) corrected energy/free energy values, respectively. Box: schematic plot of the crossing point (CP) between 2 5 and 4 5′ as well as their vertical transition species 2 5 ( v ) and 4 5′ ( v ). ( b ) Calculated structures for 2 5 and 4 5′ prior to attack of cyclooctene substrate with H-atoms on the TPA ligand omitted for clarity. Full size image Table 2 Bond length and Mulliken spin density information calculated for 2 5 and 4 5′. Full size table Our assignment of 4* as the low-spin ( κ 2 -acylperoxo)iron(III) species shown in Fig. 7 makes it the first low-spin non-heme acylperoxoiron(III) complex to be characterized thus far. The ( κ 2 -acylperoxo)iron(III) unit finds precedent in the work of Furutachi and Suzuki, who reported crystal structures of non-heme iron(III)- κ 2 -peroxocarbonate and iron(III)- κ 2 -peracetate complexes [36] , [41] . The latter complexes however differ from 4* in having high-spin iron(III) centers, which may account for their greater stability. Closely related low-spin iron(III)-peroxo complexes with HOO- and t BuOO- ligands exhibit peroxo-to-iron(III) charge transfer bands that are red-shifted relative to that of 4* , with a progression that reflects the relative basicities of the three peroxides ( λ max 460 nm and p Ka=8.2 for peracetic acid versus 510 nm and 11.8 for H 2 O 2 and 580 nm and 12.3 for t BuOOH). In addition, the molar extinction coefficient ( ε M ) of 4* , deduced to be 4,000 M −1 cm −1 on the basis of the EPR and Mössbauer quantification, is two to threefold larger than those associated with closely related low-spin Fe III complexes with end-on peroxo ligands such as [Fe(TPA*)(OOH)(NCMe)] 2+ ( ε M 2,200 M −1 cm −1 ), [Fe(TPA*)(OO t Bu)(NCMe)] 2+ ( ε M 2,200 M −1 cm −1 ), and [Fe(N4Py)(OOH)] 2+ ( ε M 1,300 M −1 cm −1 ) [30] (N4Py=bis(2-pyridylmethyl)bis(2-pyridyl)methylamine). The large ε M for 4* may arise from the postulated bidentate coordination for the acylperoxo ligand, which would enhance overlap between the metal and ligand orbitals involved in the charge transfer transition. Intermediate 4* has been trapped in the Fe II (TPA*)/H 2 O 2 /AcOH system and identified by a combination of EPR, Mössbauer, resonance Raman and ESI-MS methods to be a low-spin acylperoxoiron(III) species ( 4* ), and not an oxoiron(V) complex as proposed by Talsi [21] . Intermediate 4* forms at −40 °C and persists in a steady state phase, during which catalytic epoxidation is observed ( Fig. 3 ). Upon depletion of H 2 O 2 , 4* undergoes exponential decay at a rate that is unaffected by the nature and the concentration of the substrate, strongly implicating 4* decay to be the rate determining step for the epoxidation reaction. Computational results show that 2 4 converts to the computational species 2 5 by O–O bond homolysis, a unimolecular decomposition pathway corroborated by the experimentally observed near zero activation entropy for 4* decay and the absence of an AcOH/AcOD KIE. However, as our DFT results further show, 2 5 cannot readily epoxidise olefins and easily reverts to 2 4 ; therefore, 2 5 must isomerize to 4 5′ to move forward along the reaction coordinate towards substrate oxidation. Here again emerges a two-state reactivity that has been found for other iron oxidation systems [42] . We suggest that these mechanistic notions apply to other non-heme iron catalysts. Postulating 4 5′ as the oxidant is fully consistent with the reactivity associated with the Fe( S,S- PDP)/H 2 O 2 /RCO 2 H combination, particularly with Talsi’s observation that the enantioselectivity of epoxidation can be tuned by the R group on the carboxylic acid additive [9] and White’s beautiful results in the regio- and stereoselective transformations of C–H bonds in complex natural products [7] , [8] . Physical methods Ultraviolet–visible spectra were recorded on a Hewlett–Packard 8453A diode array spectrometer with samples maintained at low temperature by using a cryostat from Unisoku Scientific Instruments, Osaka. Electrospray mass spectrometry was performed on a Finnigan-MAT (San Jose, CA) LCQ ion trap instrument. The spectra of the reactive species were obtained by direct introduction of the solution of the intermediate generated at either −78 °C into the injector port of the spectrometer. The capillary heater on the instrument was turned off and the flow of the atomizing gas was increased to minimize thermal decomposition of the unstable intermediate. Product analyses were performed on a Perkin-Elmer Sigma 3 gas chromatograph (AT-1701 column, 30 m) with a flame ionization detector. Mossbauer spectra were recorded with two spectrometers, using Janis Research (Wilmington, MA) SuperVaritemp dewars that allow studies in applied magnetic fields up to 8.0 T in the temperature range from 1.5 to 200 K. Mossbauer spectral simulations were performed using the WMOSS software package (WEB Research, Minneapolis): Isomer shifts were quoted relative to Fe metal at 298 K. Perpendicular (9.63 GHz) mode X-band EPR spectra were recorded on a Bruker EPP 300 spectrometer equipped with an oxford ESR 910 liquid helium cryostat and an Oxford temperature controller. The quantification of the signals was relative to a Cu-EDTA spin standard. Software for EPR analysis was provided by Dr Michael P. Hendrich of Carnegie Mellon University. 1 H and 13 C NMR spectra were recorded on a Bruker Avance 500 spectrometer. Materials All reagents were purchased from Aldrich and used as received unless otherwise indicated. Preparation and handling of air-sensitive materials were carried out under an inert atmosphere by using either standard Schlenk and vacuum line techniques or a glove box. The organic substrates were purified either by passing through silical gel or by vacuum distillation before use. The Fe II (TPA) complex ( 1 ) was prepared according to published literature procedures [31] . Preparation of Fe II (TPA*) 1* The Fe II (TPA*) complex 1 * was prepared by a procedure similar to that for Fe II (TPA), where an equimolar mixture of Fe II (CH 3 CN) 2 (OTf) 2 (OTf=trifluoromethanesulfonate) and TPA* ligand in THF were stirred for 3 h (TPA*=tris(3,5-dimethyl-4-methoxypyridylmethyl)amine). Slow vapour diffusion of diethyl ether into the reaction mixture at room temperature afforded white crystals of the target product in analytically pure form. This complex was characterized via 1 H NMR and ESI-MS, while its purity was established via elemental analysis perfomed by Atlantic Microlab (Norcross, GA). Anal. Calcd (Found) for C 31 H 41 F 6 FeN 4 O 9.5 S 2 0.5 diethyl ether; C, 43.57(43.51); H, 4.64(4.83); N, 6.67(6.55) 1 H NMR (CD 3 CN, 22 °C), δ: 2.10 (br, 3H), 2.19 (br, 3H), 3.76 (br, 3H), 5.75 (br, 2H), 10.01 (br, 1H). 13 C NMR (CD 3 CN, 22 °C), δ: 13.0, 14.7, 61.9, 64.9, 128.9, 135.2, 157.9, 159.3, 167.4 ESI-MS (CH 3 CN solution) positive mode, m / z =669.1611, calculated for C 28 H 36 F 3 FeN 4 O 6 S, 669.1651. Reactivity studies Reactivity studies for the reactive intermediates were conducted under nitrogen atmosphere and were monitored via ultraviolet–visible spectroscopy at −40 °C. In a typical experiment, a 1.0 mM solution of the (L)Fe II complex in CH 3 CN (with or without AcOH) was treated with the oxidant. Upon maximum formation of the intermediate, a CH 3 CN solution of the organic substrate was added and the ultraviolet–visible chromophore of interest was monitored. In other sets of experiments, the oxidant was added to a CH 3 CN of the (L)Fe II complex in the presence of the substrate at −40 °C. Catalytic oxidations In a typical reaction carried out at 25 °C, 2 ml of a CH 3 CN solution of 1.0 mM 1* and 1.0 M of the organic substrate was prepared under aerobic conditions. The reaction was initiated by the addition of 10 eq. H 2 O 2 via syringe pump over a period of 30 min. In reactions conducted in the presence of AcOH, the additive was added prior to the addition of H 2 O 2 . At the end of the reaction, the reaction mixture was stirred for an additional 30 min after which it was worked up analysed by gas chromatography according to published procedures [15] . DFT calculations on the reaction mechanism The spin-unrestricted B3LYP functional was employed with two basis sets: (a) TZVP basis set for iron, electron-rich N and O atoms, and 6-31G** basis set for the rest C and H atoms. This basis set is denoted as B1, and was used to optimize transition states and minima; (b) The Def2-TZVPP basis set for all atoms, denoted as B2, was used for single-point energy corrections. Transition states were ascertained by vibrational frequency analysis to possess a single mode along the reaction path with only one imaginary frequency. Intrinsic reaction coordinate searching was performed to confirm transition states linking right intermediates in the 4→5/5′ conversion and cyclooctene epoxidation. All optimizations and single point calculations were performed with solvation included using the self-consistent reaction field calculations, in the polarizable continuum model; the experimental solvent acetonitrile ( ε =35.688) was used. DFT calculations were performed with Gaussian 09 suite of quantum chemical packages. How to cite this article: Oloo, W. N. et al. Identification a low-spin acylperoxoiron(III) intermediate in bio-inspired non-heme iron-catalysed oxidations. Nat. Commun. 5:3046 doi: 10.1038/ncomms4046 (2014).